A graphene field-effect transistor as a molecule-specific probe of DNA nucleobases Fast and reliable DNA sequencing is a long-standing target in biomedical research. Recent advances in graphene-based electrical sensors have demonstrated their unprecedented sensitivity to adsorbed molecules, which holds great promise for label-free DNA sequencing technology. To date, the proposed sequencing approaches rely on the ability of graphene electric devices to probe molecular-specific interactions with a graphene surface. Here we experimentally demonstrate the use of graphene field-effect transistors (GFETs) as probes of the presence of a layer of individual DNA nucleobases adsorbed on the graphene surface. We show that GFETs are able to measure distinct coverage-dependent conductance signatures upon adsorption of the four different DNA nucleobases; a result that can be attributed to the formation of an interface dipole field. Comparison between experimental GFET results and synchrotron-based material analysis allowed prediction of the ultimate device sensitivity, and assessment of the feasibility of single nucleobase sensing with graphene. Efforts to determine the order of the four nucleobases in a strand of DNA have been advancing at an extremely rapid pace in recent years [1] , [2] . Next-generation DNA sequencing technologies promise to provide cheap and high-throughput analysis of a complete DNA strand and achieve reduced sequencing artefacts. Electrical sequencing using graphene and nanopore technologies has recently attracted great attention due to the possibility to provide real-time sequencing of a whole single DNA molecule [3] , [4] , [5] , [6] , [7] , [8] , [9] , [10] , [11] . These methods are based on the use of graphene as an electrical readout-based chemical sensor while a strand of DNA is fed through a nanopore [2] , [3] , [4] , [10] . Most of the graphene-based sequencing technologies are fundamentally reliant on detecting molecular-specific interactions of individual nucleobases with a graphene surface [4] or its defects [5] . Ultimately, these interactions need to induce electronic modifications that are detectable by graphene electrical devices. Although the interaction of DNA nucleobases with graphene have been studied theoretically using molecular dynamics simulation and density functional theory (DFT) methods [12] , [13] , [14] , [15] , [16] , the experimental evidence of such specific interaction in electrical transport within the graphene has not yet been demonstrated. Graphene-based electrical sensors have already demonstrated exceptional sensor characteristics by being capable of detection of adsorption and desorption of individual gas molecules from the graphene surface [17] . This sensitivity is a direct consequence of the two-dimensional crystal structure, unique electronic properties [17] , [18] and exceptionally low-noise intrinsic characteristics of graphene based devices [19] , [20] . So far, however, single-molecule sensitivity has been reported only for nitrogen dioxide [17] , and it is not clear whether graphene can also detect other molecules, which do not induce strong charge transfer doping to graphene, down to the single-molecule level. Despite the high sensitivity of graphene devices, a key practical aspect of any chemical sensor is also their ability to distinguish between target analytes, in this case the nucleobases. Recent research has used graphene chemically functionalized with specific chemical binding groups to achieve analyte specificity [21] , [22] . Chemical functionalization, however, comes at the cost of decreased graphene mobility [23] and increased distance between the sensor and analytes, potentially hampering sensitivity. For these reasons a direct analyte–sensor interaction may be favourable for chemical sensing of individual DNA nucleobases. This leads to an important and fundamental question—can graphene detect and identify each of the nucleobases on its surface based on their specific graphene–molecule interaction. Understanding how these nucleobase–graphene interactions manifest in electric transport will be of key importance for the next-generation graphene-based DNA sequencing technologies. Here we investigate the effects of molecular adsorption of submonolayer coverages of individual DNA nucleobases on the graphene electronic structure using electric transport measurements. We demonstrate that graphene field-effect transistors (GFETs) are capable of detecting distinct coverage-dependent conductance signatures upon adsorption of the four different DNA nucleobases: adenine, guanine, cytosine and thymine. We examine the correlation between adsorption-induced nucleobase dipoles and electron transport as a function of molecular coverage and analyse the implications for single-molecule detection and identification. Furthermore, using simultaneous synchrotron-based X-ray photoelectron spectroscopy (XPS) measurements we explore the molecule-specific limit of adsorbed dipole-induced doping in a range of graphene materials. We analyse the sensitivity of our GFET devices and provide an estimate for the resolution limit in realistic scaled-down devices. Device fabrication and measurements GFET sensors, shown schematically and optically in Fig. 1 , were constructed from single-layer graphene (SLG) channels 50 μm wide and 50–200 μm long sitting on top of a SiO 2 on doped Si transistor gate. The channels were designed to be significantly larger than the common chemical vapour deposition (CVD) graphene grain size (5–10 μm 2 ) to ensure our results reflect the bulk properties of these polycrystalline graphene sheets, averaging out the effects of a range of defects present in the layers. XPS measurements were made on large area graphene samples (25 mm 2 ) fabricated identically to GFET devices but without evaporated electrical contacts. The GFET channels are comparable in size to the X-ray spot area of 50 × 100 μm 2 , allowing for reasonable comparison between the two techniques. All measurements were conducted at the Australian Synchrotron on the Soft X-ray beam line in an ultra-high vacuum (UHV) setup with base pressure <1 × 10 −9 mbar to suppress the influence of contaminating molecules adsorbed on the surface. Since water [24] and other airborne contaminants [25] have been shown to interact strongly with graphene on SiO 2 substrates, samples were thoroughly annealed after insertion into UHV. Deposition of the molecules on graphene utilized in situ low-temperature effusion cells loaded with a pure powders of the DNA nucleobases (Methods). 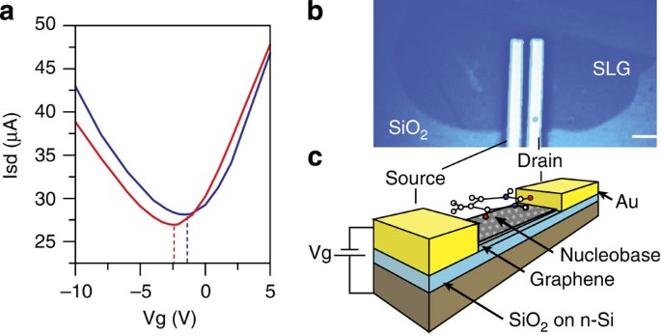Figure 1: Two terminal graphene devices used to monitor molecule-induced graphene properties. (a) Source drain current at a constant source drain voltage (10 mV) with varying gate voltage for clean (blue) graphene and 0.1 ML guanine (G) covered (red) graphene. (b) Optical and (c) schematic images of a GFET device used for electrical experiments and adsorption of each of four DNA nucleobases on graphene. Positive gate voltage is defined as a positive potential at the doped Si contact. The scale bar shown inbis 200 μm. Figure 1: Two terminal graphene devices used to monitor molecule-induced graphene properties. ( a ) Source drain current at a constant source drain voltage (10 mV) with varying gate voltage for clean (blue) graphene and 0.1 ML guanine (G) covered (red) graphene. ( b ) Optical and ( c ) schematic images of a GFET device used for electrical experiments and adsorption of each of four DNA nucleobases on graphene. Positive gate voltage is defined as a positive potential at the doped Si contact. The scale bar shown in b is 200 μm. Full size image The interaction of nucleobases with graphene was monitored with two independent measurements, via electric transport and with core level XPS. Electric transport measurements were obtained by setting a constant voltage between the source and drain contacts ( V SD ) and monitoring the source drain current ( I SD ), while the gate voltage ( V G ) was swept from −12 to 12 V. Carbon and nitrogen 1s core level (C 1s and N 1s) spectra were taken with 330 and 450 eV X-ray photons to attain high surface sensitivity and large photoionization cross section. Molecular coverage was controlled by incremental deposition and determined by comparing the ratio between the molecular N 1s peak area to the SLG C 1s peak area (Methods). Finally, we conducted angular resolved C and N K-edge near edge X-ray adsorption fine structure (NEXAFS) measurements to investigate the molecular orientation with respect to the graphene surface. Extensive beam damage studies revealed that under repeated X-ray exposure the graphene C 1s peak would shift. To ensure this effect did not interfere with any molecule-induced shifts each new XPS measurement was done on a previously unmeasured spot of the graphene sample. This also precluded direct XPS measurement of the GFET devices. Probing molecule-specific interactions Figure 1 shows a typical result of electric transport of a cleaned graphene GFET and after exposure to one of the nucleobases. The GFET spectra of all four DNA nucleobases can be found in Supplementary Information ( Supplementary Fig. 1 ). Figure 1a clearly demonstrates the high sensitivity of GFETs to adsorption of a small number of molecules, in this case ~0.1 monolayer (≈10 9 molecules) of guanine. The conductivity spectrum of graphene shifts to the left after guanine adsorption, indicating an effective n-type doping of graphene in response to adsorption of the molecules. The voltage shift of the spectra can be determined by the position of the current minima (marked by the dashed lines). The gate voltage corresponding to the minimum in I SD , known as the charge neutrality point (CNP), represents the Dirac point in the graphene band structure. The number of charge carriers in graphene is calculated using a parallel plate capacitor approximation of the doped Si/Si0 2 /graphene stack. This gives n = C BG V / e =2.46 × 10 11 cm −2 V −1 V G , where for a SiO 2 dielectric layer with and a thickness of d =90 nm. For the case of G in Fig. 1 , a 0.7 V shift indicates a relative increase of 1.7 × 10 11 electrons cm −2 in the conduction band of graphene. In Fig. 2 , we compare the induced charge carrier density in the graphene (determined from CNP shift) by adsorption of different DNA nucleobases as a function of molecular coverage. The observed coverage dependence is clearly molecule specific; however, for each molecule it can be divided into two similar regimes. In the very low coverage regime the induced charge scales approximately linearly with coverage (linear fits are displayed as dashed lines in Fig. 2 ). As the coverage increases the induced charge per molecule tails off to saturation, where adding additional molecules induces no further charge carriers. This coverage dependence is fitted by solid lines using an electrostatic depolarization model (equation 2), which attributes the observed shifts to the interface electric field formation from molecular dipoles. The depolarization model predicts the observed linearity at low coverages, and this has been experimentally confirmed for coverage-dependent work function shifts, which are also described by this model [26] , [27] . 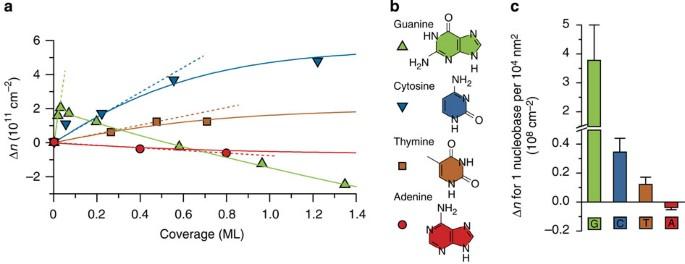Figure 2: Adsorbed nucleobase dependence of induced GFET CNP shifts. (a) Charge carrier density change (Δn) of GFETs induced by adsorption of guanine (G), cytosine (C), adenine (A) and thymine (T). The dashed lines represent linear fits to the low coverage regime used to calculate the expected single-molecule-induced shifts in (b). The solid lines are fits to C, A and T data using the electrostatic depolarization model (equation 2). The solid line for G is a guide to the eye only. (c) Calculated charge carrier density shifts of our GFETs induced by 1 nucleobase molecule per 104nm2of graphene. Figure 2: Adsorbed nucleobase dependence of induced GFET CNP shifts. ( a ) Charge carrier density change (Δ n ) of GFETs induced by adsorption of guanine (G), cytosine (C), adenine (A) and thymine (T). The dashed lines represent linear fits to the low coverage regime used to calculate the expected single-molecule-induced shifts in ( b ). The solid lines are fits to C, A and T data using the electrostatic depolarization model (equation 2). The solid line for G is a guide to the eye only. ( c ) Calculated charge carrier density shifts of our GFETs induced by 1 nucleobase molecule per 10 4 nm 2 of graphene. Full size image To assess the potential of bulk graphene devices for DNA sequencing, we have used the observed linear behaviour in the low coverage regime to extrapolate the response of GFET devices to the adsorption of single DNA nucleobase molecules, when scaling down the active sensor area. Figure 2c shows the expected change in carrier density from a single nucleobase on a GFET with 100 × 100 nm 2 of exposed graphene calculated from the linear fit to the low coverage dependence. Transport properties of GFETs of this size are still expected to be dominated by the bulk properties of graphene. The predicted induced charge carrier density in the scaled-down GFETs by the individual nucleobases is of the order of Δ n =10 6 –10 8 e, with the largest signal for adsorbed guanine showing an increase of Δ n =3.8 × 10 8 e. Even though carrier density changes in graphene of this magnitude (10 8 e) have previously been experimentally detected on larger GFETs with a device area of 1 μm 2 (ref. 17 ), the predicted signals are well below the observed noise level of our simple devices (Δ n =10 10 e). It is important to point out that these calculated signals apply to our sensors operating in a UHV environment. In ambient conditions or in a buffered ion solution where actual DNA sensors operate this sensitivity may not be achievable. An option to improve GFET sensitivity to single nucleobases is to further scale down to the graphene nanoribbon regime. Shrinking the channel area, however, increases the expected low-frequency device noise, making nucleobase signal detection more challenging. For nanoribbon devices, with devices areas of 2,000–4,000 nm 2 , noise amplitudes of the order of 10 −6 A have been reported [28] , [29] . Moreover, the electron transport in graphene nanoribbons has been shown to be dominated by edge and quantum confinement effects [30] . Another way to achieve single-molecule resolution is to improve the sensitivity of GFET devices by using a different detection method or mechanism. For instance, monitoring changes in I SD at a fixed V G is expected to significantly improve the device sensitivity in high-mobility graphene devices, because the measured signal becomes a function of the graphene charge carrier mobility ( μ ) with Δ I SD = μ G e Δ n (ref. 31 ). The recent advances in the production of high-mobility graphene devices, reaching mobility up to ≈2 × 10 5 cm 2 V −1 s −1 (refs 32 , 33 ) and the reduction of graphene device noise [34] promise to provide an improvement in device sensitivity of three orders of magnitude. This would be sufficient to detect single guanine, cytosine and thymine on 100 × 100 nm 2 GFET devices. To sense adenine, however, an additional enhancement of the sensitivity would be required. This suggests that realistic DNA sequencing with GFET devices will require use of graphene nanoribbon devices, which might exhibit completely different response to the adsorption of DNA nucleobases than our bulk GFETs because of the existence of edge states [30] , [35] . The precise control of graphene edges will be extremely important in graphene nanoribbon FETs [35] but, as recent theoretical work predicts [4] , there is a hope that 1-nm wide graphene nanoribbons with perfect arm chair edges would be able to discriminate the individual nucleobases and their sequence when a DNA strand is translocated across the ribbon. Comparison between electric transport and XPS To get a more detailed insight into the sensing mechanism of GFETs and the related molecule–graphene interactions, we have conducted, simultaneously with the electrical transport measurements, synchrotron-based XPS and NEXAFS measurements. Both of these highly surface-sensitive techniques have the capability of resolving chemical state information and conformation of adsorbed molecules on the graphene surface, information that is necessary for studying molecular adsorption processes on the atomically thin graphene samples. In addition, XPS analysis allows us to directly corroborate the measured changes in electrical data with respect to the changes in binding energy of the core level C 1s XPS peak of graphene, and thus changes in its Fermi level [36] . This was possible because the C 1s peak of graphene is well separated from the molecular C 1s peaks ( Supplementary Fig. 2 ). To compare the magnitude of the shift between the XPS C 1s position and the charge carrier density changes (Δ n ) measured via CNP, it is convenient to convert induced carrier densities to Fermi level shifts via the tight binding model approximation of graphene’s dispersion relation near the Dirac point [37] : where the Fermi velocity v F =1.0936 × 10 6 ms −1 , as measured by cyclotron resonance [38] . To test the effect of multilayered graphene, XPS measurements were obtained on both SLG and bilayer graphene (BLG) samples, with A and T molecules on the former and C and G molecules on the latter. The comparison is shown in Fig. 3 . Although the magnitude of the measured data differs, the C 1s shifts for both BLG and SLG show a qualitatively similar trend to electrical measurements. This provides strong evidence that these observations are not unique to our electrical devices and are a result of molecule-specific interactions with the bulk graphene on SiO 2 . A comparison of the differences in the magnitude of the two measurement techniques shows the measured binding energy shifts to be consistently larger than measured CNP shifts. Unlike electrical CNP measurements of GFETs, we expect the measured C 1s shifts to be independent of any graphene contact work function alignment. This would indicate that the current choice of Ti/Au contacts is limiting the GFET sensitivity to adsorbed nucleobases. 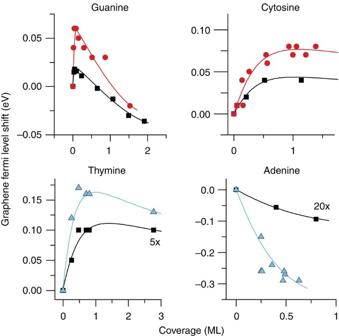Figure 3: Comparison of nucleobase-induced Fermi level shifts. Graphene Fermi level shifts of SLG GFETs (black squares) are calculated from CNP measurements using the tight binding model dispersion equation (1). XPS measurements of Fermi level shifts a determined by changes in the C 1s position of SLG (blue triangles) and BLG (red circles). The two techniques confirm the structure observed molecular coverage dependence of shifts in the graphene’s Fermi level. The error for electrical measurements was 0.005 eV, the fitting error of XPS measurements was 0.02 eV and the energy resolution of the XPS was 0.05 eV (ref.56). Figure 3: Comparison of nucleobase-induced Fermi level shifts. Graphene Fermi level shifts of SLG GFETs (black squares) are calculated from CNP measurements using the tight binding model dispersion equation (1). XPS measurements of Fermi level shifts a determined by changes in the C 1s position of SLG (blue triangles) and BLG (red circles). The two techniques confirm the structure observed molecular coverage dependence of shifts in the graphene’s Fermi level. The error for electrical measurements was 0.005 eV, the fitting error of XPS measurements was 0.02 eV and the energy resolution of the XPS was 0.05 eV (ref. 56 ). Full size image The nature of the molecular adsorption Carbon and nitrogen angle-resolved NEXAFS measurements were performed on SLG and BLG samples to obtain information about the geometry of the adsorbed molecules on graphene. NEXAFS spectra taken at a range of incident photon angles allows determination of the angle between the π * and σ * C and N orbitals and the electric field vector of the incoming light [39] . Using this technique, we observed a tilt angle of roughly 40° between each of the four nucleobases purine/pyridine rings and the graphene surface plane ( Supplementary Fig. 3 ), independent of coverage. It is important to note that this analysis could not be reliably applied to molecular coverages less than half a monolayer due to difficulties in resolving the molecular NEXAFS signal from the large graphene background. NEXAFS and XPS also allow for the direct detection of graphene–adsorbate (or substrate) hybridization [40] . No such hybridization of the graphene π * orbital was observed after nucleobase deposition on our samples, confirming that the nucleobase–graphene interaction is moderated only by van der Waals forces. This strict physisorption is important for sensors that rely on a capture sense and release mechanism, such as those previously suggested for DNA sensing [4] , [7] . The observed changes in graphene’s electronic structure on the adsorption of four individual DNA nucleobases indicate molecule-specific interactions with a strong coverage dependency. To understand whether the sensing mechanism is purely related to the molecule-induced electronic structure modification of graphene, we need to look at the molecule–graphene interface electronic structure in more detail. When a molecule is brought into contact with graphene, there are several physical effects that can influence the energy alignment of the molecular and graphene levels at the interface [41] . Previous DFT calculations of DNA nucleobases adsorbed on graphene have predicted that nucleobases interact with graphene only weakly, predominantly by van der Waals interactions [4] , [13] , [16] . The frontier molecular orbitals (highest occupied and lowest unoccupied molecular orbitals) lie far from the Fermi level of graphene [13] . As a result there is only a very weak hybridization between the molecular levels of the nucleobases and the low-lying π -states of graphene, leading to a negligible charge transfer between the molecules and graphene [13] . Even though there is almost no direct charge transfer, the electronic structure of graphene can still be significantly influenced by the molecules. It is commonly accepted that the adsorption of molecules onto a metal surface gives rise to the formation of molecular dipoles in the adsorbate layer. The effect of the electric field generated by such a dipole layer is a modulation of the surface potential of the metal, which can be measured as a change in the surface work function of the metal [26] , [27] . As graphene is a two-dimensional material the dipole electric field also modulates the number of charge carriers causing shifts in the Fermi level of the graphene, with the metal contacts acting as charge reservoirs [42] . This molecular gating is similar to the doping induced by a back gate contact when a voltage is applied. A similar mechanism has been previously reported for graphene on polymer substrates, where dipole fields of the polymer substrates caused both a work function shift and Fermi level shift in the graphene. In the case of polymer substrates, the Fermi level shift disappeared on samples without metal contacts, ruling out polymer to graphene charge transfer as the doping mechanism [43] . DFT modelling predicts that nucleobase adsorption onto graphene will also induce interfacial dipole formation, giving rise to a shift in graphene’s work function by 0.22, 0.15, 0.13 and 0.01 eV for G, A, C and T, respectively [13] . This has been calculated for one nucleobase molecule adsorbed in a flat geometry in a 5 × 5 supercell of graphene. Our experimental results, however, differ from the DFT predictions. The magnitude of measured Fermi level shifts shows a different order with respect to deposited nucleobases, and that these changes vary significantly with coverage. The consistency of our experimental shifts has been confirmed by two independent techniques and using different graphene samples from two producers. In the lower coverage regime (below 0.1 ML) the observed order of magnitude of Fermi level shift was G>C>T>A, which gradually changed to a molecular sequence of C>T>A>G at coverages greater than a monolayer. The magnitude of the shifts was in the range of 0–0.2 and 0–0.06 eV for C 1s and CNP shifts, respectively. There are several potential explanations for this strong coverage dependence and inconsistency with the previous DFT calculations. The most pointed difference being the observed angle at which the nucleobases adsorbed onto the graphene changing the strength of the molecular dipole [44] . The strong coverage dependence of DNA nucleobases induced CNP shifts in graphene can be partly explained by the aforementioned molecular gating mechanism generating shifts in CNP. The electrostatic depolarization model is commonly used to explain molecular modifications of the work function and electron affinity of semiconductor and metal surfaces due to the electric potential drop across a layer of dipolar molecules [26] , [27] . At high coverages, the mutual interaction between the formed dipole moments can lead to a strong coverage dependency [26] . This can happen with and without a direct charge transfer between molecules and substrate. The electric potential drop, which is proportional to a change in the Fermi level of graphene, can be described as a function of molecular coverage ( N ): where μ z is the z -component of the dipole moment of the molecule, α is polarizability of the molecule and c is a constant representing the geometry of the dipole lattice [26] . The fits obtained using this model to our electric transport data are shown by solid lines in Fig. 2 . The model correctly predicts an initial increase of the carrier density with increasing molecular coverage and saturation as the intermolecular interactions depolarize the absorbed molecules. The model fits well the data for C, T and A; however, the guanine data could not be properly fitted by this model due to a change of sign at high coverage. In spite of this, the depolarization model indicates quite correctly that guanine possess the highest dipole moment and polarizability, followed by C, T and A (ref. 44 ). It is important to note that the dipole moment sequence is exactly the same as the sequence observed in CNP and C 1s shifts in our experiments. The adsorption geometry of molecules is an important factor that affects the interface electronic structure. Unlike the in-plane alignment considered in most of the DFT calculations [13] , [14] , [15] , [45] , our NEXAFS measurements have shown a tilt of all four DNA nucleobases to the graphene surface of ~30–45°. The method used to calculate this tilt angle [39] , however, is sensitive to disorder in the layer, and the measured values may represent partly ordered molecular layers with patches of disordered molecules. This structure is similar to the previously observed nucleobase films on graphite by scanning tunnelling microscopy [46] , [47] . Such disorder in the molecular layers could also be caused by defects and ripples ubiquitously present in the CVD graphene samples. A different nucleobase adsorption angle on graphene is expected to significantly alter the distance between the molecules and the graphene, and the hybridization of the molecular orbitals with the graphene. Ahmed et al . [16] have recently demonstrated using DFT that the local density of states of DNA nucleobases on graphene exhibits a strong angle dependence for the molecular states within an energy range of a few electronvolts of the Fermi level. These states could be at the origin of the different sequence of nucleobase-induced shifts in our experiments compared with DFT calculations. Another possibility for the difference is the interaction of DNA nucleobases with defects in graphene or even the SiO 2 substrate. Structural defects and surface contamination are known to produce localized electronic states close to the Fermi level and act as internal or external scattering centres for electron waves, greatly degrading transport properties of graphene [48] , [49] . CVD graphene contains a range of defects, such as grain boundaries and point defects [49] . Unfortunately, the exact type of defects, the electronic structure and the nature of interactions between these graphene defects and adsorbed DNA molecules is still unknown. Although defects may play a dominant role in the observed shifts, we can exclude that a unique defect or a contamination in our samples is responsible for the sensing mechanism by observing the same results on two different graphene samples from different sources. The SiO 2 substrate can also play an important role in the sensing mechanism of GFETs on SiO 2 as has been proposed recently [50] . Using DFT modelling it has been suggested that the sensitivity of graphene to gas adsorbates can be attributed to external defects in the insulating substrate [50] . However, at this point it is difficult to clearly identify the role of these defects in our measurements and further studies are needed to elucidate the dominant sensing mechanism in our GFET devices. Although both electric transport and XPS measurements have shown qualitatively similar behaviour, there is a difference in the information obtained by these two methods. The magnitude of the observed C 1s binding energy shifts relative to Fermi level shifts calculated from CNP shifts has shown to be consistently higher for the same coverage of an adsorbed nucleobase. For instance, the C 1s shifts for thymine are five times larger than the effective shifts calculated from the electric transport using equation (1) ( Fig. 3 ). The simplest explanation for this difference is the presence of metal contacts near the measured graphene in the GFETs. Metal–graphene interfaces have been identified to have a significant influence on the transport measurements in graphene electronic devices [51] , [52] . The alignment between the metal work function (4.3 and 4.7 eV for Ti and Au) and graphene (4.5 eV) can lead to the presence of potential steps around graphene/metal contacts that have been reported to extend up to a few micrometres from the metal electrodes [52] . The contacts can thus act as effective transport barriers, causing high resistance in GFET devices. As the measured GFET transport properties are dominated by the areas of highest resistance, molecule-induced changes in the contact resistance could dominate our observed results, despite the large device areas. This characteristic indicates that if proper metal contacts are made with an optimal alignment with graphene, the electrical transport can become substantially more sensitive than seen with our graphene devices. If the measured signals from XPS are taken as the upper bound, we can expect an improvement in the sensitivity of GFETs to DNA nucleobases by up to a factor of 10 with proper metal contact engineering. While these results confirm the fundamental sensitivity of graphene for DNA sensing, the task of implementing this design of graphene sensor into any realizable DNA sequencing technology presents even further challenges not yet discussed. Water-induced doping of graphene on SiO 2 reduces device sensitivity and increases device noise [53] . As DNA sequencing is necessarily carried out in buffered ionic solutions, reduction of this effect becomes vital. Recent research has shown that using a different substrate will modify the graphene–water interactions [24] , [54] , suggesting that optimized substrate management may provide a pathway to water-based DNA sensing. Another problem faced by the use of large area graphene sensors for DNA detection is the requirement to distinguish between the effects of adsorbed nucleobases and the charged phosphate backbone. Experiments that test DNA strand sensing will be vital in understanding any phosphate backbone graphene interactions. Moreover, the device sensitivity will be influenced by the nucleobase adsorption angle that modulates the strength of the adsorbed molecular dipoles, potentially resulting in a significant difference between free nucleobases compared with attached nucleobase in a DNA strand. The charge state of graphene may provide an effective tool for electrical control of the nucleobase–graphene angle and the conformation of the DNA strand [55] . In conclusion, we have shown that the electric transport measurements using GFETs fabricated on SiO 2 can probe distinct conductance signatures upon adsorption of four different DNA nucleobases. By decreasing the size of the graphene channel in these devices and taking advantage of recent improvements in graphene mobility and noise reduction techniques, we predict that single-molecule sensing of guanine, cytosine and thymine by bulk graphene devices can be achieved. Successful device designs will require the identification and deeper characterization of dominant sensing mechanisms, combined with optimized metal contact engineering, to amplify the sensitivity of graphene devices to individual molecules. We have also established that the different nucleobases have different magnitudes of interaction with graphene that strongly depend on molecular coverage. Further research into device design may enable this molecule discriminability to be exploited for selective nucleobase sensing. Fabrication of GFETs SLG and BLG grown by CVD on Cu and transferred to SiO 2 (90 nm)/Si substrates were obtained commercially from Graphene Laboratories Inc and ACS Materials LLC. Two suppliers were used to test the effect of different intrinsic defects and impurities in the CVD graphene samples. Repeated acetone rinsing followed by a 48-h anneal at 250 °C in pure Ar (99.999%) at atmospheric pressure was used to remove residual polymethyl methacrylate from the samples. The fabrication of GFET devices was done using a polymethyl methacrylate and oxygen plasma patterning method followed by shadow mask evaporation of gold contacts (100 nm). Each sample was divided into two regions: one for the GFET devices and the second larger region for XPS analysis. SLG samples used for XPS measurements underwent the same fabrication steps to ensure any unintentional contamination was not unique to the FETs. Once loaded into the UHV system the samples were further annealed at temperatures of 250 °C in pressures <10 −9 Torr. Annealing was continued until the measured CNP did not change more than 0.1 V between subsequent annealing steps, typically between 2 and 4 h. Deposition of DNA nucleobases Powders of pure DNA nucleobases, purchased from Sigma Aldrich, were evaporated from commercial low-temperature effusion cells (MBE Komonenten) under UHV conditions. Prior to deposition the sources of DNA nucleobases were properly degassed at 110 °C for 24 h to remove water. Evaporation of DNA nucleobases was done at 138 °C for adenine, 175 °C for cytosine, 235 °C for guanine and 124 °C for thymine at a pressure of 10 −9 mbar, corresponding to a deposition rate of ~1 monolayer per 20 min. It was found that for adenine and thymine the graphene samples needed to be kept below −50 °C to ensure deposited molecules did not rapidly desorb from the surface during sample transfer in UHV. To further ensure no water contaminated the measurements, the residual gas analysis was used to verify that the water partial pressure stayed below 1 × 10 −10 mbar during evaporation. Determination of CNP from conductivity curves The CNP was taken as the gate voltage directly corresponding to the minimum measured I SD in transport measurements. The resolution limit of this method is of the order of 0.1 V due to a broad structure of the minimum conductivity region ( Fig. 1a ). A way around this problem is to estimate the CNP by the intersection of two linear fits made in the high carrier concentration regions above and below the minimum conductivity region [31] . However, as we observed a significant asymmetry between electron and hole conductivity that increased with molecular coverage, this technique would result in calculated CNPs being a function of both Fermi level shifts and the magnitude of this asymmetry and so it was not used. The changes in the device mobility with molecular adsorption were observed to be quite complex for the different nucleobases studied. Further analysis of this asymmetry and total mobility is presented in Supplementary Fig. 4 and Supplementary Discussion . Determination of molecular coverage from XPS The fractional monolayer coverages of DNA molecules on graphene were estimated using the following ratio between the XPS peak areas of the N 1s peak corresponding to a monolayer coverage and the C 1s peak area of SLG where is a geometric factor representing the ratio of the density of molecular nitrogen atoms to graphene carbon atoms, σ is the photoionization cross section of the element at a specific photon energy taken from the NIST database ( http://srdata.nist.gov/xps/ ) and I is the intensity of photons incident on the sample at a specific photon energy. Tabled values can be found in Supplementary Table 1 . Both spectra were taken at similar photoelectron kinetic energy to ensure the analyser transmission intensity was comparable for each peak. To estimate the ratio of molecular nitrogen to graphene carbon , we used the molecular unit cell sizes of monolayer coverage of each DNA nucleobase on graphite measured by scanning tunnelling microscopy [46] , [47] . How to cite this article: Dontschuk, N. et al . A graphene field-effect transistor as a molecule-specific probe of DNA nucleobases. Nat. Commun . 6:6563 doi: 10.1038/ncomms7563 (2015).